Genome-wide association study of colorectal cancer identifies six new susceptibility loci Genetic susceptibility to colorectal cancer is caused by rare pathogenic mutations and common genetic variants that contribute to familial risk. Here we report the results of a two-stage association study with 18,299 cases of colorectal cancer and 19,656 controls, with follow-up of the most statistically significant genetic loci in 4,725 cases and 9,969 controls from two Asian consortia. We describe six new susceptibility loci reaching a genome-wide threshold of P <5.0E−08. These findings provide additional insight into the underlying biological mechanisms of colorectal cancer and demonstrate the scientific value of large consortia-based genetic epidemiology studies. The estimated lifetime risk of colorectal cancer (CRC) is 5.2% for men and 4.8% for women in the United States [1] . The narrow-sense heritability estimates based on twin and family studies of CRC range from 12 to 35% (refs 2 , 3 ). Although several genome-wide association studies (GWAS) of CRC have successfully identified common single-nucleotide polymorphisms (SNPs) associated with CRC risk [4] , [5] , [6] , [7] , [8] , [9] , [10] , [11] , [12] , [13] , [14] , [15] , [16] , [17] , [18] , [19] , [20] , [21] , a large fraction of the heritability still remains elusive [22] . Our GWAS combines data from four large CRC consortia, the Colorectal Cancer Transdisciplinary (CORECT) Study, the Colon Cancer Family Registry (CFR), the Molecular Epidemiology of Colorectal Cancer (MECC) Study and the Genetics and Epidemiology of Colorectal Cancer Consortium (GECCO) to elucidate previously undiscovered susceptibility loci for CRC. The current meta-analysis identifies novel genome-wide significant risk regions at 3p14.1, 3p22.1, 10q24.2, 12q24.12, 12q24.22 and 20q13.13. Study Populations and Population Stratification Data for this discovery analysis focuses on individuals of the European ancestral heritage from North America, Australia and Europe. 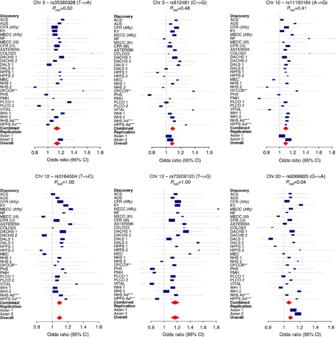Figure 1: Forest plots summarizing ORs from studies contributing to colorectal cancer meta-analysis identifying six loci reaching genome-wide significance. ThePvalue from the Cochran’sQtest for heterogeneity (Phet) is presented by SNP. ** indicates a subset of the study ARCTIC; *** indicates colorectal polyps. The study specific ORs (blue rectangles) and 95% confidence intervals (CI; horizontal bars) are plotted for each SNP. The red diamonds represent the summary OR and 95% CI for the ‘Discovery’ series (N=18,299 cases/19,656 controls) and ‘Overall’. The ‘Replication’ series included the Asian 1 (N=2,098 cases/6,172 controls) and Asian 2 (N=2,627 cases/3,797 controls) consortia. Our discovery analysis includes 19 observational studies genotyped with high-density SNP arrays and imputed to the 1,000 Genomes Project March 2012 reference panel [23] , [24] ( Supplementary Table 1 ). We employ an inverse-variance-weighted fixed-effects meta-analysis of study-specific logistic regression results after filtering data for quality control (QC). Quantile–quantile plots show no appreciable evidence of population stratification for the meta-analysis ( Supplementary Fig. 1 ) or by the individual discovery studies ( Supplementary Fig. 2 ) before and after adjustment for principal components (PCs), and the sample size-corrected marginal lambda (equivalent to 1,000 cases and 1,000 controls) measures 1.003 in the discovery meta-analysis. The PC plots for ancestry indicate no difference between cases and controls in the respective discovery GWAS studies ( Supplementary Fig. 3 ). Confirmation of Prior Studies and Discovery We evaluate the quality and effectiveness of our study design and analytic methods by assessing previously reported CRC susceptibility loci. We replicate the results for 41 of the 47 ( P <0.05, unadjusted for multiple testing) published autosomal susceptibility variants for CRC ( Supplementary Table 2 ). We turn our attention to the discovery of new susceptibility loci ( Supplementary Fig. 4 ) by investigating the top 200 independent loci detected in the European discovery phase ( Supplementary Table 3 ) in two separate East Asian consortia. Overall, our combined meta-analysis across European and Asian studies discovers six new susceptibility loci reaching a statistical threshold of P <5.0E−08: at chromosome 3p22.1 (rs35360328), 3p14.1 (rs812481), 10q24.2 (rs11190164), 12q24.12 (rs7137828), 12q24.22 (rs73208120) and 20q13.13 (rs6066825; Table 1 ; Supplementary Table 4 ). The odds ratios (ORs) across these six loci indicate a range of a 9 to 16% increase in the odds of developing CRC per risk allele, similar to previously reported CRC susceptibility loci. A seventh susceptibility locus tagged by rs4946260 at 6q22.1 approaches genome-wide significance ( P =6.27E−08). The ORs are consistent across populations and genotyping platforms as shown by chi-square tests for heterogeneity, with only one locus showing marginally significant heterogeneity (rs6066825/20q13.13, P het =0.04). Table 1 Newly identified genetic susceptibility loci for colorectal cancer. Full size table Replication in Asian Populations Forest plots for the six genome-wide significant loci show that the risk alleles identified in the European populations replicate broadly across the Asian populations even though allele frequencies differ substantially ( Fig. 1 ). Two SNPs were not available for replication in the Asian studies because they are rare in Asians. Figure 1: Forest plots summarizing ORs from studies contributing to colorectal cancer meta-analysis identifying six loci reaching genome-wide significance. The P value from the Cochran’s Q test for heterogeneity ( P het ) is presented by SNP. ** indicates a subset of the study ARCTIC; *** indicates colorectal polyps. The study specific ORs (blue rectangles) and 95% confidence intervals (CI; horizontal bars) are plotted for each SNP. The red diamonds represent the summary OR and 95% CI for the ‘Discovery’ series ( N =18,299 cases/19,656 controls) and ‘Overall’. The ‘Replication’ series included the Asian 1 ( N =2,098 cases/6,172 controls) and Asian 2 ( N =2,627 cases/3,797 controls) consortia. Full size image Genomic Location and Candidate Genes Several of the six susceptibility SNPs fall within regions harbouring genes known to be involved in the pathogenesis of CRC ( Supplementary Fig. 5 ). Rs35360328 and a corresponding tagSNP at 3p22.1 (rs35364139, r 2 =0.8, P =1.7E−07) lie in an intergenic region within ∼ 300 kb of CTNNB1 , the gene that encodes β-catenin. β-Catenin is a key member of the WNT signalling pathway and is commonly mutated in CRC development [25] , [26] . There are no histone marks in the vicinity of either rs35360328 or rs35364139 in any colon-derived cells in the publicly available ENCODE chromatin immunoprecipitation (ChIP)-seq tracks, making these unlikely to be the functional SNPs in this region ( Supplementary Fig. 5 ). However, there are 26 other SNPs in linkage disequilibrium (LD) with rs35364139 ( r 2 >0.5, CEU population), which may disrupt biofeatures or regulatory elements resulting in the observed CRC risk. Together, the physical proximity of this newly identified susceptibility locus, relevant functional biology and adjacent regulatory marks suggest that CTNNB1 is an intriguing candidate target gene of a putative enhancer. The second locus on chromosome 3 is located at 3p14.1 (rs812481) and is intronic of LRIG1 , a gene encoding a transmembrane protein that interacts with epidermal growth factor receptor-family tyrosine kinase family members [27] , [28] , [29] . LRIG1 has recently been described as a marker of quiescent colon crypt stem cells activated to proliferate following injury [30] . No histone marks are found in the vicinity of rs812481, making it unlikely to be the functional SNP. Notably, rs3856595 ( P =2.4E−07), in LD ( r 2 >0.5, CEU population) with rs812481, is located in a LRIG1 intronic active enhancer peak (H3K27ac4) in sigmoid colon epithelium. A second SNP in LD with rs812481 is rs231276 ( P =2.0E−06), which resides in an H3K4me1 enhancer peak in a CRC cell (HCT-116). This peak is intronic of SLC25A26 , a mitochondrial transport protein. The SNP at 10q24.2 (rs11190164) lies in a genomic region containing multiple genes including SLC25A28 , ENTPD7 , COX15 , CUTC and ABCC2 . Several SNPs in high LD with rs11190164 map to putative enhancers, promoters or 3′ UTRs of genes within the region. A recent study identified rs1035209, 6.3 kb upstream from rs11190164 (CEU r 2 =0.4), to be significantly associated with CRC risk [17] . In addition, rs3740078 (distance to rs11190614=93,887 bp, r 2 =0.71, CEU population; P =3.2E−05) causes a synonymous change in the coding sequence of ENTPD7 . While ENTPD7 has been linked to intestinal epithelial inflammation in mice and is expressed in normal colonic epithelium [31] , a role in CRC has not been previously reported. Rs3184504 at 12q24.12 implicates SH2B3 as a putative target gene for CRC susceptibility. SH2B3 is an adaptor protein involved in cytokine signalling and functions as a classic tumour suppressor gene in B-precursor acute lymphoblastic leukaemia that increases STAT3 phosphorylation [32] . Less is known about its signalling roles in the colon, but rs3184504 is a missense variant (Trp262Arg) that is a known risk allele for coeliac disease and other immune-related disorders [33] and is a well-established risk factor for type 1 diabetes [34] and hypertension [35] . Several other SNPs in LD with rs3184504 also map to putative regulatory regions, but further work is needed to functionally characterize this missense variant or these other SNPs. Other genes within this region, including CUX2 , BRAP and ACAD10 are also potential candidate genes. The SNP at 12q24.22 (rs73208120) is independent of rs3184504 at 12q24.12 ( r 2 =0.002, CEU population) and lies intronic of NOS1. NOS1 encodes neuronal nitric oxide synthase 1 that generates nitric oxide a reactive free radical involved in several biologic processes, including inflammation, infection and antimicrobial and antitumoral activities [36] . There are several SNPs in LD with rs73208120, but none map to the candidate enhancer regions. The SNP at 20q13.13 (rs6066825) lies within an intron of the PREX1 gene that encodes the Rac-guanine nucleotide exchange factor P-Rex1, a signalling protein involved in cell migration and invasion in some cell types [37] . There are 35 SNPs in LD with rs6066825 ( r 2 >0.5, CEU population), all intronic or immediately downstream of PREX1 . The most promising functional candidates are three SNPs, rs2092492 ( r 2 =0.62, CEU population), rs6066823 ( r 2 =0.62, CEU population) and rs6066825 itself that lie within a putative active enhancer marked by an H3K27ac ChIP-seq peak in sigmoid colon tissue. In conclusion, the combined meta-analysis of 52,649 individuals facilitated the discovery of six new susceptibility loci for CRC. Additional CRC loci remain to be discovered despite the large sample sizes included in our discovery meta-analysis. Although replication of suggestive loci from the discovery phase in similar ancestral populations would be more powerful due to LD and effect allele frequency differences, this study identified six novel CRC risk loci. This study identified opportunities to explore new biologic mechanisms for predisposition to CRC and the potential for translation into improved risk prediction for populations of diverse ancestral heritage. Our initial GWAS combined data from three large CRC consortia, the CORECT Study, the CFR, the MECC and the GECCO to elucidate previously undiscovered susceptibility loci for CRC. Data for this discovery analysis focused on individuals of European ancestral heritage from North America, Australia and Europe. Detailed methods are described in the Supplementary Methods . In brief, samples from 19 observational studies genotyped with high-density SNP arrays and imputed to the 1,000 Genomes Project March 2012 reference panel [24] contributed to the discovery meta-analysis. Replication of the top 200 independent SNPs was performed in two additional consortium studies from Asian populations. The studies included in the discovery and replication phases are listed in Supplementary Table 1 . Discovery phase genotyping and QC The details on study design and characteristics for each study and substudy in the discovery phase are provided in the Supplementary Methods . In brief, the discovery phase consisted of four CRC consortia. The CORECT consortium coordinated genotyping and analysis of six observational studies of CRC for the present analysis: (1) MECC2, (2) CFR2, (3) Kentucky case–control study, (4) American Cancer Society CPS II nested case–control study, (5) Melbourne nested case–control study and (6) Newfoundland case–control study. Genotyping as part of CORECT was conducted using a custom Affymetrix genome-wide platform (the Axiom CORECT Set) with ∼ 1.3 million SNPs and insertions and deletions (indels) on two physical genotyping chips (pegs). In the MECC1 study, germline DNA was extracted from peripheral blood samples and genotyped in two batches using the Illumina HumanOmni 2.5–8 BeadChip, which measures nearly 2.4 million SNPs and indels. Batch 1 (414 cases and 155 controls) was run at the Case Western Reserve University and batch 2 (104 cases and 376 controls) was run at the University of Michigan. Germline DNA for the CFR1 study was extracted from peripheral blood samples and genotyped in two batches using three different platforms—the Illumina Human1M or Human1M-Duo (CFR1-Set1) and the Illumina HumanOmni1-Quad (CFR1-Set 2)—each containing ∼ 1.2 million SNPs and indels. Genotype data were cleaned based on QC metrics at the individual subject and SNP levels. Samples with <95% call rate, sex mismatches (between self-reported and genotypic predicted sex), low concordance with previous genotype data, duplicate samples, unanticipated genotype concordance, identity-by-descent with another sample or ethnic outliers as identified by visual inspection of PCA cluster plots were removed. Before imputation, SNPs with <95% call rate, concordance <95% with 1000 Genomes in samples genotyped for QC, or Hardy–Weinberg equilibrium P <10 −4 in controls were excluded. All SNPs overlapping 1000 Genomes were matched to the forward strand. The GECCO consortium consists of 13 studies. Details are provided in Supplementary Methods and Supplementary Table 1 . In brief, DNA was extracted from blood samples or from buccal cells, using conventional methods. Phase one genotyping was done using either Illumina HumanHap 550K, 610K or combined Illumina 300 and 240K, Affymetrix platforms [18] , Illumina HumanCytoSNP or Illumina HumanOmniExpress. All studies included 1 to 6% blinded duplicates to monitor quality of the genotyping. All individual-level genotype data were managed and underwent QA/QC at the Ontario Institute for Cancer Research, the University of Washington or at the Fred Hutchinson Cancer Research Center. Details on the QA/QC have previously been described [12] . In brief, samples were excluded based on call rate, heterozygosity, unexpected duplicates, gender discrepancy and unexpectedly high identity-by-descent or unexpected genotype concordance (>65%) with another individual. All analyses were restricted to samples clustering with the Utah residents with Northern and Western European ancestry from the CEPH collection (CEU) population in PC analysis, including the HapMap II populations as reference. SNPs were excluded if they were triallelic, not assigned an rs number, or were reported or observed as not performing consistently across platforms. In addition, genotyped SNPs were excluded based on call rate (<98%), lack of Hardy–Weinberg equilibrium in controls ( P <1 × 10 −4 ) and minor allele frequency (MAF) (<5% in Set 1 for PLCO, WHI, DALS and OFCCR; minor allele count<10 for remaining studies). Imputation To meta-analyse genotype data generated from multiple platforms and to increase the coverage of variation that is measurable across the genome, imputation of genotypes was performed for both autosomal (all consortia) and X chromosome (excluding GECCO consortium) markers. Imputing missing genotypes for study samples based on the cosmopolitan panel of reference haplotypes from Phase I of the 1,000 Genomes Project (March 2012 release; n =1,092; ( ftp://ftp-trace.ncbi.nih.gov/1000genomes/ftp/release/20110521 )) [23] , [24] helps improve imputation accuracy of low-frequency variants [38] . The target panel was phased using Beagle [39] (GECCO) or SHAPE-IT [40] (CORECT, MECC1 and CFR1) and the phased target panel was imputed to the 1000 Genomes reference panel using either Minimac [41] (GECCO) or IMPUTE2 (ref. 42 ) (CORECT, MECC1 and CFR1). Genetic markers retained following imputation had to pass stringent imputation quality and accuracy filters before entering the analysis phase. For GECCO, Rsq was used as the imputation quality measure for imputed SNPs [43] , and SNPs were excluded at different Rsq thresholds based on their MAF: for SNPs with MAF>0.01, we excluded those with Rsq≤0.3; for MAFs of 0.005–0.01, we excluded Rsq<0.5; and for MAF<0.005, we excluded Rsq<0.99. In the remaining studies (CORECT, MECC1 and CFR1) stringent imputation quality and accuracy filters (info ≥0.7, certainty ≥0.9, concordance ≥0.9) were applied between directly measured and imputed genotypes after masking input genotypes (for genotyped markers only) to enter the analysis phase. Further, we restricted the SNP list to those with study-specific MAF≥1%. Statistical analysis We utilized PC analysis to assess correspondence between self-reported and genotypic classification of ancestry including unrelated HapMap CEU, YRI and ASN samples as population controls. Ancestral outliers were identified by visual inspection of PC plots for each study and removed. PCs were computed and used for ancestry adjustment. Study-specific association estimates (OR and 95% CI) were obtained employing logistic regression of CRC on allelic dosage adjusting for ancestry and potential confounding variables (for example, age, sex and study site) as defined by the individual studies ( Supplementary Methods ). The genomic control factor ( λ ) was estimated by dividing the median χ 2 -statistic by 0.456. A sample size-corrected marginal λ , equivalent to studying 1,000 cases and 1,000 controls, was also calculated. Heterogeneity of genetic effects by study was assessed using Cochran’s Q test for heterogeneity ( P het ). Replication phase The replication phase was conducted in two Asian consortia (Asian 1 and Asian 2). The Asian Colorectal Cancer Consortium (ACC), Asian 1, consisted of five studies with genome-wide scan data: Shanghai CRC study 1 (Shanghai-1); Shanghai CRC Study 2 (Shanghai-2); Guangzhou CRC Study (Guangzhou); Aichi CRC Study 1 (Aichi-1), and the Korean Cancer Prevention Study-II CRC (KCPS-II). Samples in these studies were genotyped using Affymetrix and Illumina SNP arrays for GWAS ( Supplementary Methods ) [10] , [44] , [45] , [46] , [47] , [48] . A uniform QC protocol (call rates, concordance rates, cryptic relatedness, sex misidentification and ancestry) to filter samples and SNPs was applied [10] . Imputation was performed with the GIANT ALL data panel from the 1,000 Genomes Project phase 1 release v3 as the reference using program MACH v1.0 (ref. 43 ) and minimac [41] . SNPs with imputation R 2 >0.7 in each of the five studies were included in the final analysis. Associations between SNPs and CRC risk were evaluated based on the log-additive model using mach2dat [43] . Per-allele ORs and 95% confidence intervals (CIs) were derived from logistic regression models, adjusting for age, sex and the first ten PCs when appropriate. Association analysis was conducted for each participating study separately and a fixed-effects meta-analysis was conducted to obtain summary results with the inverse-variance method using program METAL [49] . The Asian 2 consortium was genotyped using the Illumina 1M-duo Array and consisted of studies from the Multiethnic Cohort (MEC; N =3,094), CFR ( N =285), Colorectal cancer study on Oahu, Hawaii (CR2 & 3; N =134), Fukuoka, Japan ( N =1,411), Nagano, Japan ( N =207) and the Japan Public Health Center-based prospective study (JPHC; N =1,293) after QC filtering [50] , [51] , [52] , [53] , [54] . In general, all genotyped samples were examined and excluded according to the following: (1) call rates <90, 95 or 97% depending on the batches, (2) missing on basic covariates (age, sex or disease status), (3) gender mismatch, (4) ethnicity outliers and (5) relatedness (≥2nd degree). Prediction of untyped or partly genotyped SNPs was performed with BEAGLE 3.3 (ref. 39 ) using the 1,000 Genomes Project (phase 1, release 3) East Asians as reference panels. Imputation was performed with all cases and controls combined. Markers with MAF<0.005 in reference panels were excluded from imputation. Study-specific association statistics were obtained using logistic regression models adjusted for ancestry and potential confounding variables ( Supplementary Methods ). A fixed-effects meta-analysis was conducted to obtain summary results with the inverse-variance method using programme METAL [49] . All study samples were collected with written informed consent, and procedures were approved by the Human Research institutional review boards (IRBs) of the respective institutions. Specifically, the University of Southern California Health Sciences IRB approved all elements of the CORECT, CFR and MECC studies. The MECC study protocol was also approved by the IRBs at the University of Southern California, University of Michigan, and Carmel Medical Center (Haifa). The Fred Hutchinson Cancer Research Center IRB approved the GECCO contribution. The Asian 1 consortia study protocols were approved by the review board of the Vanderbilt University Medical Center and informed consent was obtained from all study participants. Study protocols of the Asian 2 consortia were approved by the University of Hawaii Human Studies Program and University of Southern California IRB, the IRB in the National Cancer Center, Japan and the Ethics Committee of Kyushu University Faculty of Medical Sciences. Meta-analysis A consortia-wide meta-analysis for the discovery and replication phases using fixed-effect models with inverse variance weighting was implemented in METAL. Heterogeneity was evaluated using Cochran’s Q test for heterogeneity and the measure I 2 . Graphical representation of effect estimates and CIs by study and consortia are presented using forest plots. How to cite this article: Schumacher, F. R. et al . Genome-wide association study of colorectal cancer identifies six new susceptibility loci. Nat. Commun. 6:7138 doi: 10.1038/ncomms8138 (2015).